Generation of acoustic self-bending and bottle beams by phase engineering Directing acoustic waves along curved paths is critical for applications such as ultrasound imaging, surgery and acoustic cloaking. Metamaterials can direct waves by spatially varying the material properties through which the wave propagates. However, this approach is not always feasible, particularly for acoustic applications. Here we demonstrate the generation of acoustic bottle beams in homogeneous space without using metamaterials. Instead, the sound energy flows through a three-dimensional curved shell in air leaving a close-to-zero pressure region in the middle, exhibiting the capability of circumventing obstacles. By designing the initial phase, we develop a general recipe for creating self-bending wave packets, which can set acoustic beams propagating along arbitrary prescribed convex trajectories. The measured acoustic pulling force experienced by a rigid ball placed inside such a beam confirms the pressure field of the bottle. The demonstrated acoustic bottle and self-bending beams have potential applications in medical ultrasound imaging, therapeutic ultrasound, as well as acoustic levitations and isolations. As is well known, an acoustic beam tends to propagate along a straight line and suffers broadening from diffraction in a homogeneous medium. To route acoustic waves along a curved trajectory, metamaterial-based transformation acoustics tailors the properties of the acoustic media along the trajectory of propagation, akin to the transformation optics that twists and transforms the Cartesian coordinates of electromagnetic fields [1] , [2] , [3] , [4] . Acoustic metamaterials consisting of sub-wavelength unit cells enable unprecedented material properties including negative density, negative modulus, as well as extreme anisotropy [5] , [6] , [7] , [8] , [9] , [10] , and more importantly, offer an extraordinary bending power over sound waves to realize acoustic cloaking devices [11] , [12] , [13] , [14] and super-resolution acoustic imaging [15] , [16] , [17] . However, such a control based on spatially varying material properties could be largely limited or even inhibit important applications which do not allow invasions, for example, imaging or energy delivery into a three-dimensional living biological entity behind another sensitive organ. Finding a way to bend the wave field without engineering the medium is therefore highly desirable. Here we design and synthesize acoustic beams that are capable of directing sound energy along curved paths and circumventing obstacles in an otherwise homogeneous media. Without loss of generality, we demonstrate a bottle-shaped acoustic beam ( Fig. 1 ), where the sound energy flows through a three-dimensional curved shell leaving a null-pressure region in the middle. The construction of such acoustic bottles relies on a general recipe developed here, which can route acoustic beams along arbitrary convex trajectories. Moreover, we show that the wall of the acoustic bottle exerts a pulling force on a rigid object placed inside, demonstrating its ability for acoustic trapping. The developed beam design methodology can be readily applied to other frequency regimes in different media, leading to potential applications in medical imaging [18] , therapeutic ultrasound [19] , acoustic levitations and manipulations [20] , [21] , as well as nonlinear and pulsed acoustics [22] . 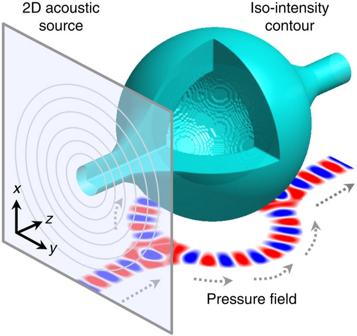Figure 1: Schematic illustration of an acoustic bottle beam. After being emitted from a planar-phased sound source, the sound energy flows through a three-dimensional curved shell in air leaving a close-to-zero pressure region in the middle, exhibiting the capability of circumventing obstacles. Here we assume that the acoustic wave propagates along thezaxis, and thexandyaxes are taken as the transverse coordinates. The evolution of the pressure field displayed at the bottom manifests the self-bending ability of the acoustic bottle beams to avoid a three-dimensional space. The dashed arrows indicate the proceeding direction of the wavefront. Figure 1: Schematic illustration of an acoustic bottle beam. After being emitted from a planar-phased sound source, the sound energy flows through a three-dimensional curved shell in air leaving a close-to-zero pressure region in the middle, exhibiting the capability of circumventing obstacles. Here we assume that the acoustic wave propagates along the z axis, and the x and y axes are taken as the transverse coordinates. The evolution of the pressure field displayed at the bottom manifests the self-bending ability of the acoustic bottle beams to avoid a three-dimensional space. The dashed arrows indicate the proceeding direction of the wavefront. Full size image Self-bending acoustic beam To produce the acoustic bottle depicted in Fig. 1 , we first develop a general recipe for self-bending acoustic beams that propagate along any prescribed arbitrary convex trajectories in a two-dimensional setting, followed by the introduction of an axial symmetry to construct the acoustic bottle beams in three dimensions. In general, self-bending beams represent exact solutions of the wave equation [23] , [24] , [25] . In a lossless and source-free homogeneous medium, the pressure p of a time-harmonic acoustic wave obeys the Helmholtz equation ∇ 2 p + k 2 p =0, where ∇ 2 is the Laplace operator, and k is the wave number. Considering a two-dimensional case, the acoustic self-bending beams propagating along any given convex trajectory x = f ( z ) can be found by solving the Helmholtz equation asymptotically [26] . Such self-bending waves can be understood as a caustic wave phenomenon, where a family of delicately arranged tilted rays coalesces onto a curved trajectory upon propagating, leaving a uniform and concentrated non-diffracting beam. Tracing each individual caustic ray allows us to measure the phase retardation and construct a specific wavefront at the acoustic source plane, which produces a self-bending beam (see Methods). By such a design methodology along with axial symmetry, the three-dimensional acoustic bottle beams can be realized. Recently, wave packets with self-bending ability have been demonstrated with laser and electron beams [27] , [28] , [29] , which has inspired a variety of applications including generating curved plasma channels [30] , synthesizing linear light bullets [31] and guiding microparticles [32] . Here, we create for the first time the self-bending acoustic beams and acoustic bottles. The self-bending acoustic wave packets identified here are able to propagate along curved trajectories in a homogeneous medium, similar to the ballistic motion of the projectile under the action of gravity. We synthesize an acoustic beam propagating along a free-form Bézier curve in air [33] by employing a planar speaker array [34] , as shown in Fig. 2 . A cubic Bézier curve is a parametric curve that can be scaled indefinitely, and in the meantime the smooth trajectory is prescribed by four control coordinates that are arbitrarily chosen (purple circles in Fig. 2a ). The wavefront (blue curves) for generating the cubic Bézier self-bending beam, as shown in Fig. 2a , can be obtained by following the acoustic rays to the source plane (see Methods). In our experiment, we launch the desired self-bending sound beams by precisely adjusting the phase retardation of a linear array of 40 speakers operating at a frequency of 10 kHz (1.5 cm in diameter with 2.5 cm spacing). As such, the phase profile of a prescribed beam can be directly imprinted onto the emitted sound waves by addressing the phase of each individual speaker. The produced acoustic field is then scanned by an acoustic transducer. 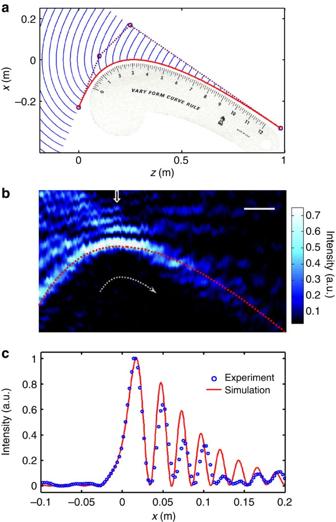Figure 2: Demonstration of a self-bending acoustic beam propagating along an arbitrary convex trajectory. (a) The predesigned beam trajectory (red) that follows a cubic Bézier curve as indicated by a varying form curve rule, where the purple circles mark the four control points of the Bézier curve, and the blue curves describe the calculated geometric wavefront. (b) Experimentally measured acoustic intensity distribution of the generated Bézier self-bending beam following the design in (a), where the red dashed curve indicates the predesigned trajectory, the grey dashed curve indicates the propagation direction of the beam; scale bar, 0.1 m. (c) The transverse acoustic intensity profile taken along the white vertical arrow inb(crossing the apex of the trajectory), showing a good agreement between experiment (blue circles) and theory (red curve). a.u., arbitrary unit. Figure 2b displays a self-bending acoustic beam with an asymmetric transverse beam profile ( Fig. 2c ), which indeed follows the designed Bézier curve and is able to circumvent obstacles. It is also observed that the diffraction of the self-bending beam is largely suppressed in comparison with a Gaussian beam of similar beam size (see Methods). Moreover, due to its caustic nature, such a self-bending acoustic wave packet is extremely robust against perturbations. It even reconstructs its beam structure after encountering obstacles during propagation. To demonstrate the self-reconstructing behaviour of the self-bending acoustic beam, we inserted a steel rod as an obstacle with a diameter of 3.75 cm (grey disk in Fig. 3 ) into the beam path to block the main lobe of the beam. The corresponding numerical simulation ( Fig. 3a ) and the experimental result ( Fig. 3b ) clearly indicate that the self-bending acoustic beam indeed can restore the beam structure after the main lobe is blocked. Such a self-reconstruction property is critical in practice, especially in applications such as acoustic imaging and therapeutic ultrasound through heavily scattering and inhomogeneous media. Figure 2: Demonstration of a self-bending acoustic beam propagating along an arbitrary convex trajectory. ( a ) The predesigned beam trajectory (red) that follows a cubic Bézier curve as indicated by a varying form curve rule, where the purple circles mark the four control points of the Bézier curve, and the blue curves describe the calculated geometric wavefront. ( b ) Experimentally measured acoustic intensity distribution of the generated Bézier self-bending beam following the design in ( a ), where the red dashed curve indicates the predesigned trajectory, the grey dashed curve indicates the propagation direction of the beam; scale bar, 0.1 m. ( c ) The transverse acoustic intensity profile taken along the white vertical arrow in b (crossing the apex of the trajectory), showing a good agreement between experiment (blue circles) and theory (red curve). a.u., arbitrary unit. 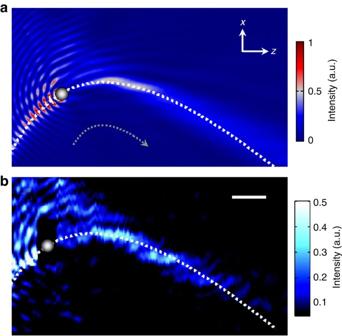Figure 3: Self-reconstruction of self-bending acoustic beams. Numerical simulation (a) and experimental measurement (b) demonstrate that the synthesized self-bending acoustic beam propagating along a cubic Bézier curve (white dashed line) is capable of reconstructing its beam profile after the main lobe is blocked by a steel rod (grey disk) in the beam path. The grey dashed arrow inaindicates the proceeding direction of the acoustic beam. Scale bar, 0.1 m. a.u., arbitrary unit. Full size image Figure 3: Self-reconstruction of self-bending acoustic beams. Numerical simulation ( a ) and experimental measurement ( b ) demonstrate that the synthesized self-bending acoustic beam propagating along a cubic Bézier curve (white dashed line) is capable of reconstructing its beam profile after the main lobe is blocked by a steel rod (grey disk) in the beam path. The grey dashed arrow in a indicates the proceeding direction of the acoustic beam. Scale bar, 0.1 m. a.u., arbitrary unit. Full size image Acoustic bottle beam and acoustic pulling force By rotating the self-bending beam structure, we can create an acoustic bottle beam, which encloses a region with close-to-zero sound pressure surrounded by a higher acoustic pressure shell in three dimensions ( Fig. 1 ). We used the discretized speaker array as shown in Fig. 4a with designed amplitude and phase profile (see Methods). The measured axial cross-section and transverse beam profiles of the acoustic field of the bottle beam show that the sound beam emitted from the planar source creates a transversely localized forward propagating wave packet before the beam expands into a ring and follows along a curved path ( Fig. 4b–h ). Such curved propagation behaviour of the wave packet can be further confirmed and visualized by our full-wave numerical simulations ( Fig. 4i , also see Methods). As a matter of fact, the shape and size of the three-dimensional bottle can be controlled at ease because the self-bending trajectory can be engineered to an arbitrary convex trajectory as demonstrated above. Moreover, if there is an object residing in the ‘dark’ region of the acoustic bottle, it will largely remain unperturbed from the acoustic energy, and in return does not perturb the propagation of the beam. The dynamics of such behaviours can be clearly visualized in Supplementary Movie 1 . The capability of the acoustic bottle to circumvent obstacles relies on the interference of the sound waves. Therefore it relies on the coherence of the acoustic fields in the medium, which is in stark contrast to the acoustic invisibility devices relying on the spatially varying medium. 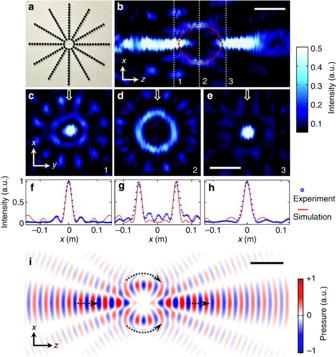Figure 4: Production of an acoustic bottle beam in three dimensions. (a) The speaker array used in our experiment (1.5 cm diameter and with a radial spacing 2.5 cm). (b–e) Measured acoustic intensity maps of the axial cross-section (b) and the transverse cross sections (c–e) at different longitudinal positions as marked inb, where the predesigned bottle profile is marked by the red dashed lines. (f–h) The acoustic intensity profiles taken along the white vertical arrows inc–e(crossing the beam center), respectively, showing a good agreement between experiment (blue circles) and theory (red line). (i) Numerical simulations of the axial cross-section of the pressure field of the designed acoustic bottle beam, where the dashed arrows indicate that the sound energy indeed flows through the curved shell of the bottle. The animation of the pressure field of the bottle beam and a comparing Gaussian beam (Supplementary Movie 1) shows the self-bending dynamics and the capability of circumventing obstacles of the acoustic bottle field. Scale bar, 0.1 m. a.u., arbitrary unit. Figure 4: Production of an acoustic bottle beam in three dimensions. ( a ) The speaker array used in our experiment (1.5 cm diameter and with a radial spacing 2.5 cm). ( b – e ) Measured acoustic intensity maps of the axial cross-section ( b ) and the transverse cross sections ( c – e ) at different longitudinal positions as marked in b , where the predesigned bottle profile is marked by the red dashed lines. ( f – h ) The acoustic intensity profiles taken along the white vertical arrows in c – e (crossing the beam center), respectively, showing a good agreement between experiment (blue circles) and theory (red line). ( i ) Numerical simulations of the axial cross-section of the pressure field of the designed acoustic bottle beam, where the dashed arrows indicate that the sound energy indeed flows through the curved shell of the bottle. The animation of the pressure field of the bottle beam and a comparing Gaussian beam ( Supplementary Movie 1 ) shows the self-bending dynamics and the capability of circumventing obstacles of the acoustic bottle field. Scale bar, 0.1 m. a.u., arbitrary unit. Full size image As shown in Supplementary Movie 1 , when a rigid object resides in the acoustic bottle, it experiences a minimal scattering of acoustic field. When the object is gradually moving out of the ‘dark’ region, the bottle field will be severely disturbed. Such scattering of the wave field will inevitably give rise to the acoustic radiation force for confining the objects within the ‘bottle’ [35] . In fact, radiation-force-based acoustic levitation and tweezers by conventional acoustic beams have been well studied [20] , [21] . To experimentally test the possibility of trapping via an acoustic bottle beam, we directly measure the acoustic radiation force along the axial axis using a rigid ball made of a hard plastic material ( Fig. 5a ). When the rigid ball resides in the bottle, the axial radiation force can be negative, indicating the existence of a pulling force against the beam propagation direction as well as the gravity ( Fig. 5c ). In contrast, when the rigid sphere is out of the ‘dark’ region, a strong pushing force along the propagation direction is observed. Such a pulling/pushing force is originated from the scattering of the sphere (see the vicinity of the boundary indicated by the blue dashed circle in Fig. 5b ). The measured acoustic radiation force can be numerically calculated by solving the vector surface integral of the radiation-stress tensor (defined as the time average of the wave momentum flux) over a surface enclosing the object (blue dashed circle in Fig. 5b ) [35] . The theoretical results (red curve) are in good agreement with the experimental data. The achieved force in our experiment is relatively weak (~μN) due to the poor speaker efficiency in our experiment (~0.1% at the maximum electrical power 0.5 W for each speaker). Much stronger acoustic forces can be expected by simply employing higher-power acoustic sources to generate bottle beams for acoustic trapping, imaging and therapeutic purposes. Note that the acoustic loss in our current experiment is negligible (~4% per metre). When extending our method into different environment and frequency ranges where the loss and inhomogeneity of the medium are much larger, one should take into account these factors when solving the wave equation. 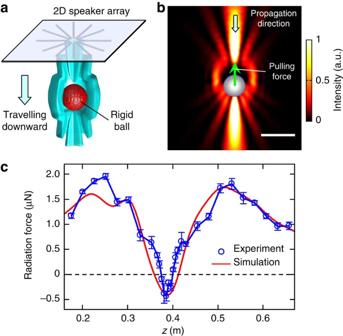Figure 5: Acoustic pulling force originated from the acoustic bottle beam. (a) Schematic of the setup used for measuring the acoustic radiation force with a rigid hard plastic ball. (b) Calculated acoustic intensity of the bottle beam in the presence of the rigid ball (corresponding to the positionz=0.383 inc), where the stronger scattering at the bottom indicates the origination of a pulling force; scale bar, 0.1 m. (c) Experimentally measured (blue data points) and numerically simulated (red curve) acoustic radiation forces of the bottle beam at different axial locations, where the region below the dashed line incindicates the existence of the acoustic pulling forces in the opposite direction of the beam propagation as well as the gravity. The error bar depicts the standard deviation of our measurement. a.u., arbitrary unit. Figure 5: Acoustic pulling force originated from the acoustic bottle beam. ( a ) Schematic of the setup used for measuring the acoustic radiation force with a rigid hard plastic ball. ( b ) Calculated acoustic intensity of the bottle beam in the presence of the rigid ball (corresponding to the position z =0.383 in c ), where the stronger scattering at the bottom indicates the origination of a pulling force; scale bar, 0.1 m. ( c ) Experimentally measured (blue data points) and numerically simulated (red curve) acoustic radiation forces of the bottle beam at different axial locations, where the region below the dashed line in c indicates the existence of the acoustic pulling forces in the opposite direction of the beam propagation as well as the gravity. The error bar depicts the standard deviation of our measurement. a.u., arbitrary unit. Full size image We demonstrated a method of routing acoustic waves along designed arbitrary curved paths in homogeneous media. This offers a new degree of freedom for controlling the flow of acoustic energy at will [4] , [5] , [6] , [7] , [8] , [9] , [10] , [11] , [12] , [13] , [14] , [15] , [16] , [17] , [18] , [36] . We further demonstrated an acoustic bottle beam capable of trapping. Such an approach opens a new avenue for diffractionless acoustic beam routing [37] that is important for applications such as underwater sonar and ultrasound medical imaging that need to access the hard-to-reach objects hidden behind obstacles. Theoretical formulation of self-bending acoustic beams In a lossless and source-free homogeneous medium, the pressure p of a time-harmonic acoustic wave is governed by the Helmholtz equation where ∇ 2 is the Laplace operator, k =2π f / c s is the wave number, and c s and f denote the speed and frequency of the sound, respectively. For a one-dimensional case, assuming that a wave packet propagates in the x – z plane, equation (1) becomes Here we take the x and z as the transverse and longitudinal coordinates, respectively. Previous studies have shown that self-bending (or self-accelerating) beams can be found by solving the wave equation (equation (2)) [23] , [24] , [25] . Such a beam, after being launched from a plane source at a certain position (for example, z =0), shall maintain its beam profile and suffer a transverse shift along the x axis while proceeding in the z direction. Due to the fact that exact solutions of equation (2) are only available for certain limited coordinate systems [23] , [24] , [25] , identifying the self-bending beam along an arbitrary trajectory is a nontrivial issue. As is well known, the asymptotic theory provides an efficient way to construct the solution of partial differential equations [26] . It has been shown that the solution of equation (2) can be presented in the form of asymptotic series [26] , [38] , [39] where the phase function ψ and the amplitude functions A j are complex. By substituting equation (3) into equation (2), we can find that ψ satisfies the eikonal equation of geometrical acoustics [39] whereas A j satisfies the recursive system of transport equations where j =0,1,2,…, and A −1 ≡0. The solution of equation (4) describes the geometric wavefront as well as the rays, which determine the propagation of the amplitude governed by equation (5). Such decoupled condition offers us the opportunity to construct the rays and the successive positions of the wavefront without any reference to the amplitude of the self-bending beams. This can be easily understood in terms of Huygens’ Principle. Our recipe is to construct a self-bending beam as the asymptotic solution of equation (2) by finding the wavefront determined by the predesigned trajectory of the self-bending beam from equation (4), without referencing to the amplitude distribution. From a mathematical point of view, the field constructed in such a way is the leading part of the asymptotic expansion of the exact field. Although the full asymptotic expansion consists of additional terms in the amplitude of the field on each ray, these terms are much smaller than the first term [38] , [39] . This is equivalent to the approximation made in the ray acoustics theory, from which it has been shown that quite accurate results can be reached even at a scale that is close to the sound wavelength [39] . As pointed out in previous studies, the self-bending beam represents an envelope of rays and there exists a singular gradient mapping between the ray surface (wavefront) and the self-bending beams (caustics) [23] . As shown in Fig. 6 , the geometric representation of such a condition is that all the rays forming a caustic are tangents of the caustic trajectory. As the geometric wavefront is always perpendicular to the rays, one can construct a unique wavefront family from the tangential rays of the caustic trajectory. Once the wavefront is determined, the phase map on a planar source plane can be generated by tracing each point on the wavefront to the source plane along the ray and calculating the phase retardation [28] . To formulate our recipe, let us consider a phased array located in x – z plane emitting acoustic rays according to a certain phase profile φ ( x ), as illustrated in Fig. 6 . During the propagation along the positive z axis, the rays construct a desired self-bending wave packet at x = f ( z ), where the single-valued function f depicts an arbitrary convex curve. Next we shall use Legendre transformations to construct the geometric wavefront from a preset beam trajectory. 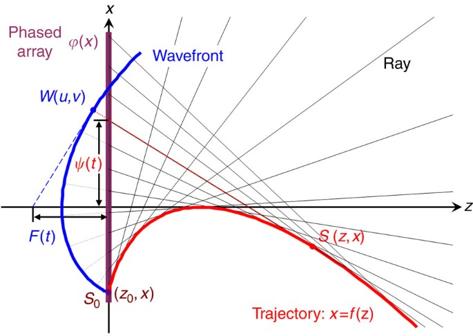Figure 6: Asymptotic theory of self-bending acoustic beams. The rays (thin black lines) emitted from the wavefront (blue curve) construct a caustic (red curve), creating a self-bending acoustic beam. Each ray is being a tangent of the trajectory. The phase modulation of the phased array (thick magenta line) is directly derived from the wavefront. Figure 6: Asymptotic theory of self-bending acoustic beams. The rays (thin black lines) emitted from the wavefront (blue curve) construct a caustic (red curve), creating a self-bending acoustic beam. Each ray is being a tangent of the trajectory. The phase modulation of the phased array (thick magenta line) is directly derived from the wavefront. Full size image Assume that the geometric wavefront W corresponding to an arbitrary convex beam trajectory S can be described by the parametric curve ( u ( x , z ), v ( x , z )). The Legendre transformation of S can be written as From Fig. 6 , one can easily derive that Therefore the Legendre transformation of W can be written as From equations (8) and (10), we obtain By applying inverse Legendre transformation, we can obtain where ψ is a function of t . Solving equation (13) with the method of variation of constants, we obtain where C ( z 0 ) is a fixed constant for a certain S 0 at z 0 . Then from equations (11) and (12), we arrive at Considering t = f′ ( z ) and S 0 is the intersection point of W and S , equation (15) turns into To construct the phase profile for the planar-phased array from the curved wavefront described by equation (16), one needs to trace each point on a wavefront along the ray to the plane of phased array and calculate the phase retardation. This gives the phase profile for creating the acoustic self-accelerating beam along the predesigned curve f ( z ), which is determined by the following parametric equations By solving equations (16) and (17) for a given desired beam trajectory, one can readily construct the phase profile needed for the phase array. Notice that there is no approximation involved in the above phase profile construction process, and therefore our recipe remains accurate for highly non-paraxial condition [28] . Design of the self-bending Bézier beam To demonstrate the feasibility of our recipe for designing acoustic self-bending beams, here we chose a Bézier curve as a typical example [33] . A Bézier curve is a parametric curve P ( t ), which is a polynomial function of the parameter t . The curve is defined by a set of control points P 0 through P n , where n is called its order ( n =1 for linear, 2 for quadratic, and so on.). An explicit definition of a Bézier curve of degree n can be expressed as In our experiment, we chose a cubic ( n =3) Bézier curve, which is defined by four points P 0 , P 1 , P 2 , P 3 and is expressed as a cubic polynomial By substituting equation (19) into equations (16) and (17), we can calculate the phase profile required for creating acoustic self-bending beams travelling along the cubic Bézier trajectory, as shown in Fig. 7a . By discretizing the phase profile according to our speaker arrangement (see Fig. 7b ), we can readily obtain the phase retardation of each speaker (see Fig. 7a ). 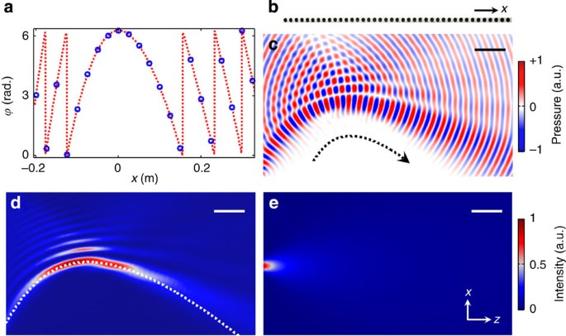Figure 7: Generation of a self-bending acoustic beam along a Bézier curve. (a) The wrapped phase profile for synthesizing the Bézier beam, where the red dashed line represents the profile obtained from the theory and the blue data points correspond to the modulations applied onto the speaker array. (b) The speaker array consisting 40 speakers (1.5 cm in diameter and 2.5 cm spacing) used in our experiment. (c–d) Numerically simulated sound pressure and intensity of the generated beam. (e) The propagation of an input Gaussian beam with a similar beam size of the main lobe of the Bézier beam ind. Scale bar, 0.1 m. a.u., arbitrary unit. Figure 7c,d depict the numerical simulations of the generated acoustic pressure field (c) and the intensity distribution (d) from the phase profile, where the black dashed arrow indicates the beam propagation direction, whereas the white dashed line denotes the predesigned trajectory. The pressure field shown in Fig. 7c clearly indicates that the generated beam indeed propagates along the predesigned Bézier curve. In comparison with the propagation of a Gaussian beam at similar beam size, the diffraction of the generated self-bending Bézier beam is largely suppressed. Note that the spacing between the adjacent speakers in our array (2.5 cm) is larger than half of the sound wavelength at 10 kHz (~1.72 cm), which will cause the spatial aliasing effect [40] . However, our numerical simulations and experimental results show that such an effect is only observable in the region close to our speaker array and near the edge of the array. Figure 7: Generation of a self-bending acoustic beam along a Bézier curve. ( a ) The wrapped phase profile for synthesizing the Bézier beam, where the red dashed line represents the profile obtained from the theory and the blue data points correspond to the modulations applied onto the speaker array. ( b ) The speaker array consisting 40 speakers (1.5 cm in diameter and 2.5 cm spacing) used in our experiment. ( c – d ) Numerically simulated sound pressure and intensity of the generated beam. ( e ) The propagation of an input Gaussian beam with a similar beam size of the main lobe of the Bézier beam in d . Scale bar, 0.1 m. a.u., arbitrary unit. Full size image Construction and modelling of speaker array In our experiment, the phase and the amplitude profiles of the acoustic wave emitted from the speaker array (see Fig. 7b ) are controlled by a home-built all-pass filter array and an audio amplifier array, respectively. A simple first-order all-pass filter can generate a phase delay of Δ φ =180°−2arctan(2π fRC ) without changing the amplitude of the signal. Here f is the signal frequency, R is the control resistor and C is the control capacitor of the all-pass filter. For each speaker, we used one first-order all-pass filter to achieve a phase delay from 0° to 180°, or two first-order all-pass filters connected in series to achieve a phase delay from 180° to 360°. We generated the desired phase delays (see Fig. 7a ) by changing the values of tunable resistors (a typical value: 0–50 kΩ) whereas the capacitors possess fixed values (typically at 1 nF). The audio amplifiers used in the experiment are TDA7052A/AT made by Philips Semiconductors, which has a maximum output of about 1 W. Numerical simulations of the speaker array are carried out using the acoustics module of Comsol Multiphysics. In our Comsol simulation, we use the ‘plane wave’ radiation boundary condition that assigns a uniform pressure value over the whole area of each speaker. This is equivalent to approximate the speaker as a superposition of many equally-distributed dipoles, which represents the experimental system better than a simple monopole or dipole approximation [34] . The pressure amplitude and phase of the source are defined separately. All the speakers are arranged periodically along one straight boundary, and all other boundaries are set at the scattering boundary condition. Methodology of designing and generating acoustic bottle beams To generate acoustic bottle beams with different three-dimensional shapes, we circularly wrap the self-bending beam with respect to the z axis, as illustrated in Fig. 8a . Specifically, we wrap the self-bending beam with respect to a point (named as a singular point) residing on the beam trajectory. As such, one can derive an axial symmetric wavefront according to the one-to-one mapping between the rays and the bottle boundary in the transverse (critical) plane containing the singular point. Consequently, the phase profile at the critical plane can be obtained with equations (16) and (17). As indicated from Fig. 8a , to the left beyond the singular point, the one-to-one mapping will abruptly disappear. Next, we address how to create acoustic bottle beams from a source that is placed at a certain position located on the negative z axis beyond the critical plane. Due to the lack of the one-to-one mapping from bottle structure to the phase map, one has to involve modulations in both amplitude and the phase. Suppose the source is placed at z =− z 0 , the required phase and amplitude can be deduced from the phase map at the critical plane via a backward propagating process. 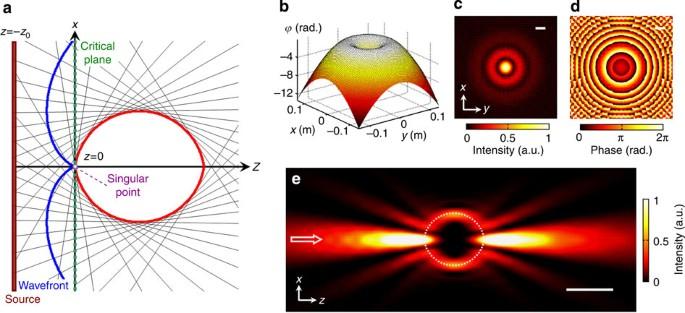Figure 8: Design methodology of acoustic bottle beams. (a) Illustration of the method. (b–e) Numerical simulation results. As shown ina, from the one-to-one mapping between the rays (thin black lines) and the boundary of the bottle beam (red curve) at the critical plane (z=0, except the singular point), we first construct the wavefront (blue curve) and then the pure phase map (b) at the critical plane (vertical dashed line). With a backward propagating process, we can obtain the amplitude (c) and phase modulation (d) required for the production of the designed bottle beam atz=−z0, the intensity cross-section of which is shown ine, where the white dashed curves depict the predesigned bottle shape. Scale bar, 0.1 m. a.u., arbitrary unit. By employing the angular spectrum theory, the back propagation of an acoustic field p ( x ,0) can be described by [41] Figure 8: Design methodology of acoustic bottle beams. ( a ) Illustration of the method. ( b – e ) Numerical simulation results. As shown in a , from the one-to-one mapping between the rays (thin black lines) and the boundary of the bottle beam (red curve) at the critical plane ( z =0, except the singular point), we first construct the wavefront (blue curve) and then the pure phase map ( b ) at the critical plane (vertical dashed line). With a backward propagating process, we can obtain the amplitude ( c ) and phase modulation ( d ) required for the production of the designed bottle beam at z =− z 0 , the intensity cross-section of which is shown in e , where the white dashed curves depict the predesigned bottle shape. Scale bar, 0.1 m. a.u., arbitrary unit. Full size image where F {} and F −1 {} represent Fourier transform and inversed Fourier transform, respectively. Figure 8b–d show an example of the back propagation procedure for generating a bottle beam by wrapping up a self-bending beam with respect to the origin ( x = z =0). The circular trajectory of the self-bending beam is described by . Figure 8b displays the phase map at the critical plane constructed from equations (16) and (17). The amplitude and phase profile obtained by the backward propagation for generating bottle beams from a planar source (located at z =−0.36) are shown in Fig. 8c,d , respectively. The axial intensity cross-section of the generated bottle beam from numerical simulation is displayed in Fig. 8e , from which it can be seen that the generated bottle beam matches the initial design well. As it can be seen, inside the bottle there is no sound energy. This means if we put any obstacle inside the bottle, it would not influence the beam propagation at all. Such a behaviour is clearly illustrated in Supplementary Movie 1 . To experimentally generate the bottom beam shown in Fig. 8 , we utilize the speaker arrangement as shown in Fig. 9a . The required amplitude and phase modulation for the axial symmetrically arranged speakers are plotted in Fig. 9b . The amplitude profile shown in Fig. 9b was calculated on the basis of the assumption that the speakers were distributed uniformly. In the experiment, the spacing of speakers increases along the azimuth direction. So we set the amplitude of each speaker equal to the calculated amplitude shown in Fig. 9b multiplied by a factor that is proportional to the radius of the circle where the speaker is located. The numerical simulations with such an arrangement are shown in Fig. 9c–f , from which we can clearly see that a bottle structure has been successfully generated. 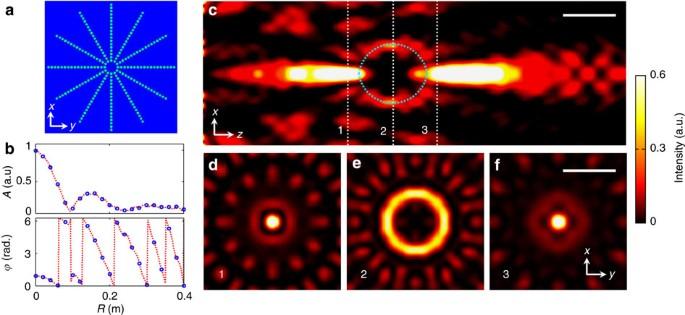Figure 9: Simulated performance of the designed speaker array. (a) Arrangement of the speaker array in our experiment. (b) Amplitude (top) and phase (bottom) of the radial modulation of the speaker array, where the red dashed line represents the profile obtained from the theory and the blue data points correspond to the modulations applied onto the speaker array. (c–f) Numerical simulations of the longitudinal (c) and transverse (d–f) intensity distributions of the generated bottle beam, where the turquoise dashed curves incdepict the predesigned bottle shape. Scale bar, 0.1 m. a.u., arbitrary unit. Figure 9: Simulated performance of the designed speaker array. ( a ) Arrangement of the speaker array in our experiment. ( b ) Amplitude (top) and phase (bottom) of the radial modulation of the speaker array, where the red dashed line represents the profile obtained from the theory and the blue data points correspond to the modulations applied onto the speaker array. ( c – f ) Numerical simulations of the longitudinal ( c ) and transverse ( d – f ) intensity distributions of the generated bottle beam, where the turquoise dashed curves in c depict the predesigned bottle shape. Scale bar, 0.1 m. a.u., arbitrary unit. Full size image Acoustic field mapping method All experiments are conducted with a system similar to the one used in our previous work under room temperature inside a large room to isolate the ambient noise and air flow [42] . The generated acoustic fields from the speaker arrays are mapped by measuring the sound pressure amplitude with a 4-mm diameter PUI Audio TOM-1045S-C33-R microphone. Under our measurement condition, the acoustic intensity map can be derived from the pressure measurement by I = p 2 / Z 0 = p 2 /413, where a purely real acoustic impedance of air Z 0 =413 N s m −3 is used by assuming that the sound pressure and particle velocity are in phase within our measured region. To minimize the field perturbations from the measurement, the microphone is attached to a thin metal holder, which is mounted onto a three-dimensional motor controlled scanning system and runs in a zigzag way to cover the whole field. All the measured data were sent to a computer through Tektronix TDS2002B digital storage oscilloscope for further processing. Both three-dimensional motor controlled scanning system and TDS2002B were controlled by LabVIEW software. Characterization of acoustic radiation force The radiation force exerted on an object by a continuous-wave surface acoustic wave can be obtained by solving the vector surface integral of the radiation-stress tensor (defined as the time average of the wave momentum flux) over a surface enclosing the object [35] . Within the second-order approximation, the acoustic radiation force can be governed by [35] , [43] where S is a fixed surface enclosing the object, ρ and c s are the fluid density and speed of sound, p and v are the acoustic pressure and particle velocity, n is the outward normal to the surface S , dS is the elementary surface element, and the angular bracket <·> denotes the time average. To quantify the radiation force of the acoustic bottle beams exerted on an object, we performed numerical simulation with the acoustics module of Comsol Multiphysics. By placing the object at different locations in the acoustic field and choosing S to be the boundary surface of the object, the acoustic field under perturbation of the object was first simulated with Comsol, and then the acoustic radiation force was calculated according to equation (21). To experimentally measure the acoustic radiation force of the bottle beam exerting on an object, the speaker array emitting a downward propagating beam is placed on the top. The force is probed in air by a rigid ball made of hard plastics (6.5 cm in diameter). The rigid ball is supported by a very thin rigid rod (1 mm in diameter), which is connected to a digital analytical scale with a reading accuracy of 0.01 mg. By measuring the weight difference in the presence and absence of the acoustic field at different locations, the acoustic radiation force of the bottle field can be mapped out. We repeated the measurement many times by turning on and off the acoustic source about every 30 seconds, and then took the average of the results to increase the accuracy of the measurement. The setup was placed in a sealed box to avoid air turbulence, and the walls of the box were covered by foam to reduce the sound reflection. To prevent the acoustic wave directly hitting on the analytical scale, we utilized a very long thin rod for connecting the rigid ball and covered the analytical scale with a plate and foam. The relative longitudinal position between the two-dimensional speaker array and the analytical scale are precisely adjusted by a vertical translation system. How to cite this article: Zhang, P. et al . Generation of acoustic self-bending and bottle beams by phase engineering. Nat. Commun. 5:4316 doi: 10.1038/ncomms5316 (2014).